Metastasis-associated protein 1 is an integral component of the circadian molecular machinery The mammalian circadian clock regulates the daily cycles of many important physiological processes, but its mechanism is not well understood. Here we provide genetic and biochemical evidence that metastasis-associated protein 1 (MTA1), a widely upregulated gene product in human cancers, is an integral component of the circadian molecular machinery. Knockout of MTA1 in mice disrupts the free-running period of circadian rhythms under constant light and normal entrainment of behaviour to 12-h-light/12-h-dark cycles. The CLOCK–BMAL1 heterodimer activates MTA1 transcription through a conserved E-box element at its promoter. MTA1, in turn, interacts with and recruits CLOCK–BMAL1 at its own and CRY1 promoters and promotes their transcription. Moreover, MTA1 deacetylates BMAL1 at lysine 538 through regulating deacetylase SIRT1 expression, thus disturbing the CRY1-mediated negative feedback loop. These findings uncover a previously unappreciated role for MTA1 in maintenance of circadian rhythmicity through acting on the positive limb of the clock machinery. The mammal circadian clock is a complex physiological process that results in generating about 24-h rhythms in organism behaviour, metabolism and other functions [1] . The proposed mechanism for circadian rhythmicity is composed of a set of autoregulatory transcription/translation feedback loops that have both positive and negative arms [1] , [2] , [3] . At the positive arm, the transcriptional factors CLOCK and BMAL1 form a heterodimer and drive the transcription of the cryptochrome ( CRY ) and period ( PER ) genes through binding to the E-box elements present in their promoters [3] , [4] , [5] . Once PER and CRY proteins reach a critical concentration, they interact to form complexes with CLOCK–BMAL1 and repress their own transcription, thus acting as negative components of the circadian feedback loops [2] , [6] , [7] . Eventually, removal of the PER-CRY repressor complex through, at least in part, the ubiquitin-dependent degradation depresses CLOCK–BMAL1 activity, thus initiating a new cycle [8] , [9] , [10] , [11] . Despite these advances, our understanding of the intrinsic mechanism for driving the mammalian circadian clock remains rudimentary. Since its identification by differential complementary DNA library screening using the 13762NF rat mammary adenocarcinoma metastatic system [12] , the metastasis-associated protein 1 (MTA1) has evolved into an important marker for human cancers [13] . In this context, MTA1 is upregulated in a wide variety of human cancers and its expression levels are closely correlated with tumour aggressiveness and metastasis [13] . MTA1 was subsequently identified as a key component of the nucleosome remodelling and histone deacetylase (HDAC; NuRD) complex [14] , [15] , thus establishing MTA1 as a transcriptional corepressor via covalent modification of histones [16] . Interestingly, the NuRD-independent mechanisms for MTA1 in regulating the expression of genes such as BCAS3 , ARF and PAX5 are now being recognized [17] , [18] , [19] . In addition to its overexpression in cancer cells and tissues, MTA1 is detected in most of the normal mouse tissues with significant levels present in the brain, lung, ovary, mammary gland and testis [20] , [21] , but its normal physiological functions in development and other biological processes are not well understood. Here we provide the evidence that MTA1 has a physiologically important role in orchestrating the circadian clock via regulating the CLOCK–BMAL1 heterodimer-driven feedback loops. In this context, MTA1 is a clock-controlled gene that is transcriptionally activated by CLOCK–BMAL1. In turn, MTA1 associates with CLOCK–BMAL1 and regulates its own transcription and CRY1 gene expression mediated by CLOCK–BMAL1. Moreover, MTA1 deacetylates BMAL1 at lysine 538 by regulating deacetylase SIRT1 expression, and the MTA1-SIRT1-BMAL1 deacetylation axis is required for transcriptional activation of MTA1 and CRY1 by CLOCK–BMAL1. MTA1 knockout results in abnormal circadian behaviour in mice During analyzing the mouse MTA1 promoter sequence, we recognized the presence of a canonical E-box motif (5′-CACGTG-3′) [4] , [5] , [7] and two non-canonical E-box motifs (5′-CAGCTT-3′) [22] within 5-kbp promoter region in the MTA1 promoter ( Supplementary Table S1 ). In contrast, the closely related MTA2 and MTA3 genes contain a non-canonical E-box motif (5′-CAGCTT-3′) in their promoters ( Supplementary Table S1 ). Further, the canonical E-box motif present in the MTA1 promoter is highly conserved among multiple species including human, monkey, chicken, dog and cow ( Supplementary Table S2 ). Given that E-box regulatory elements are the common hallmark of the promoters of clock-controlled genes in mammals [23] , we reasoned that MTA1 may exert a previously unappreciated physiological function in the mammalian circadian clock. To test this possibility, we first examined whether genetic depletion of MTA1 influences the circadian behaviour in an in vivo physiological setting by comparing wheel-running activity, the benchmark assay for circadian dysfunction [24] , of wild-type (MTA1 +/+ ) and MTA1-knockout (MTA1 −/− ) mice in constant darkness (DD) or constant light (LL) after prior entrainment to a 12-h-light/12-h-dark (12/12 LD) cycle for 3 weeks [25] ( Fig. 1a ). As shown in Fig. 1b , there was no difference in the free-running period under DD ( τ DD) between MTA1 +/+ and MTA1 −/− mice (23.6±0.3 versus 23.5±0.3 h, mean±s.d., P =0.07; Student’s t -test). In contrast, the free-running period in LL ( τ LL) was longer in MTA1 −/− mice (25.3±0.7 h; mean±s.d.) than that in wild-type animals (24.9±0.2 h, mean±s.d. ; P <0.05; Student’s t- test). Moreover, the change in the free-running period (Δ τ ) after switching to LL was greater in MTA1 −/− mice (1.9±0.8 h, mean±s.d.) than that in wild-type counterparts (1.2±0.4 h, mean±s.d., P <0.01; Student’s t -test). These findings reveal a role for MTA1 in regulating the response of the circadian clock to ambient light. 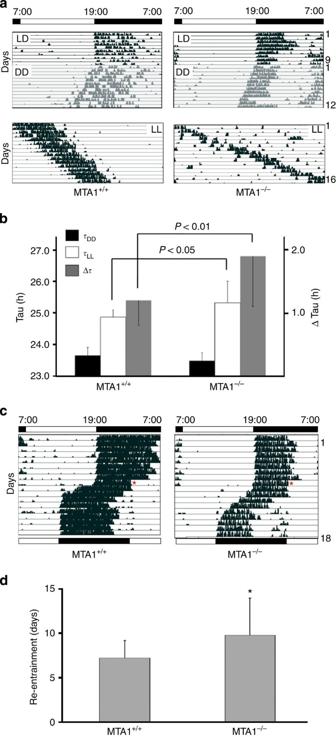Figure 1: Loss of MTA1 resulted in altered circadian wheel-running behaviour in mice. (a) Representative actograms of MTA1+/+and MTA1−/−mice. All animals were housed individually in cages equipped with running wheels. After at least 3 weeks under a LD cycle consisting of 12 h of light (150 lux) followed by 12 h of darkness (<0.01 lux), mice were remained in DD or LL (150 lux) for at least 4 weeks. A grey background indicates the dark periods and the bar above the activity record shows the LD cycle. The horizontal bars above each actogram indicate the lighting condition (open=150 lux; filled=darkness). Top panels show actograms of mice maintained under LD12:12, then switched to DD (shaded area). Bottom panels show actograms from animals maintained under constant light (LL; 150 lux). (b)τwas determined by Periodogram analysis of 400 continuous hours of wheel-running data collected from animals maintained under DD or LL. Values represent the mean±s.d. of 15 MTA1+/+(12 males and 3 females) and 17 MTA1−/−(13 males and 4 females) mice forτDD, of 12 MTA1+/+(9 males and 3 females) and 10 MTA1−/−(7 males and 3 females) mice forτLL and Δτ. Filled bars=τDD; open bars=τLL; shaded bars=Δτ(τLL−τDD). The free-running period in LL (τLL) was significantly longer (0.4 h;P<0.05; two-tailed Student’st-test) in MTA1−/−mice than that in MTA1+/+mice. In addition, the change in the free-running period (Δτ) after switching to LL was significantly greater (58%;P<0.01; pairedt-test) in MTA1−/−mice. (c) Representative actograms from MTA1+/+and MTA1−/−mice. The LD cycle was shifted forward at the time indicated by the red asterisks, resulting in a 6-h truncation of the prior dark phase. The horizontal bars indicate the lighting conditions (open=150 lux; filled=darkness) either before (above the actograms) or after (below the actograms) the 6-h advance. (d) Values represent the mean±s.d. of 15 MTA1+/+(12 males and 3 females) and 16 MTA1−/−(12 males and 4 females) mice. Asterisk *P<0.05; two-tailed Student’st-test. Figure 1: Loss of MTA1 resulted in altered circadian wheel-running behaviour in mice. ( a ) Representative actograms of MTA1 +/+ and MTA1 −/− mice. All animals were housed individually in cages equipped with running wheels. After at least 3 weeks under a LD cycle consisting of 12 h of light (150 lux) followed by 12 h of darkness (<0.01 lux), mice were remained in DD or LL (150 lux) for at least 4 weeks. A grey background indicates the dark periods and the bar above the activity record shows the LD cycle. The horizontal bars above each actogram indicate the lighting condition (open=150 lux; filled=darkness). Top panels show actograms of mice maintained under LD12:12, then switched to DD (shaded area). Bottom panels show actograms from animals maintained under constant light (LL; 150 lux). ( b ) τ was determined by Periodogram analysis of 400 continuous hours of wheel-running data collected from animals maintained under DD or LL. Values represent the mean±s.d. of 15 MTA1 +/+ (12 males and 3 females) and 17 MTA1 −/− (13 males and 4 females) mice for τ DD, of 12 MTA1 +/+ (9 males and 3 females) and 10 MTA1 −/− (7 males and 3 females) mice for τ LL and Δ τ . Filled bars= τ DD; open bars= τ LL; shaded bars=Δ τ ( τ LL−τDD). The free-running period in LL ( τ LL) was significantly longer (0.4 h; P <0.05; two-tailed Student’s t -test) in MTA1 −/− mice than that in MTA1 +/+ mice. In addition, the change in the free-running period (Δ τ ) after switching to LL was significantly greater (58%; P <0.01; paired t -test) in MTA1 −/− mice. ( c ) Representative actograms from MTA1 +/+ and MTA1 −/− mice. The LD cycle was shifted forward at the time indicated by the red asterisks, resulting in a 6-h truncation of the prior dark phase. The horizontal bars indicate the lighting conditions (open=150 lux; filled=darkness) either before (above the actograms) or after (below the actograms) the 6-h advance. ( d ) Values represent the mean±s.d. of 15 MTA1 +/+ (12 males and 3 females) and 16 MTA1 −/− (12 males and 4 females) mice. Asterisk * P <0.05; two-tailed Student’s t -test. Full size image We next examined whether disruption of MTA1 affects entrainment of mice to the light-dark (LD) cycles, another fundamental property of circadian rhythmicity [26] ( Fig. 1c ). In this context, mice entrained to a 12/12 LD cycle were subjected to light-phase advancement by 6 h and the re-entrainment of locomotor activity was compared between MTA1 +/+ and MTA1 −/− mice ( Fig. 1c ). Interestingly, MTA1 −/− mice took 9.8±4.2 (mean±s.d.) days to fully adapt to the new LD cycle, whereas MTA1 +/+ mice adapted substantially faster, taking 7.2±2.0 (mean±s.d.) days to reach full re-entrainment ( Fig. 1d , P <0.05; Student’s t -test). Together, these results provide the first genetic evidence that MTA1 is essential for the generation and maintenance of circadian rhythms under constant light and for normal entrainment of behaviour to LD cycles. MTA1 depletion disrupts circadian expression of clock genes As a serum shock induces circadian gene expression in mammalian cells [27] , we next examined whether the levels of MTA1 protein and messenger RNA exhibit rhythmic changes in the wild-type mouse embryonic fibroblasts (MEFs) following serum shock at different time points. Using the core clock proteins CLOCK and BMAL1 as positive controls, we demonstrated that a serum shock induces MTA1 protein expression in MTA1 +/+ MEFs in a circadian manner ( Fig. 2a ). Consistently, oscillatory expression of MTA1 mRNA was also observed in serum-shocked MTA1 +/+ MEFs ( Fig. 2b ). We next examined whether knockout of MTA1 affects the rhythmic expression of MTA2 and MTA3 genes and core clock genes in serum-shocked MTA1 +/+ and MTA1 −/− MEFs. Interestingly, MTA2 and MTA3 exhibited rhythmic expression in MTA1 +/+ MEFs following serum shock in a circadian manner ( Fig. 2d and e ). Although MTA1 knockout did not affect the levels of MTA2 and MTA3 proteins ( Fig. 2c ), it altered the circadian patterns of MTA2 ( Fig. 2d ) and MTA3 expression ( Fig. 2e ) in the MTA1 −/− MEFs following serum shock. In addition, the expression patterns of the endogenous core clock genes including CLOCK ( Fig. 2f ), BMAL1 ( Fig. 2g ), CRY1 ( Fig. 2h ), CRY2 ( Fig. 2i ), PER1 ( Fig. 2j ), PER2 ( Fig. 2k ) and SIRT1 ( Fig. 2l ) were disrupted in the MTA1 −/− MEFs as compared with its levels in the MTA1 +/+ cells following serum shock. These results support the notion that MTA1 is an integral component of the clock machinery. 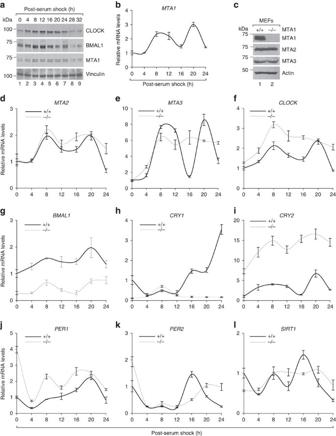Figure 2: Depletion of MTA1 disrupts the rhythmic expression of core clock genes. (a,b) MTA1+/+MEFs were grown to confluence in DMEM/F-12 medium containing 5% fetal bovine serum (FBS) for 6 days and shifted to medium containing 50% adult horse serum for 2 h. At time=0, the serum-rich medium was replaced with serum-free medium and cells were collected at the indicated time points for western blot analysis with the indicated antibodies (a) or qPCR analysis ofMTA1mRNA levels (b). (c) Protein extracts from MTA1+/+and MTA1−/−MEFs were subjected to the western blot analyses with the indicated antibodies. (d–l) Serum-shocked MTA1+/+and MTA1−/−MEFs as described above were collected at the indicated time points for qPCR analysis ofMTA2(d),MTA3(e),CLOCK(f),BMAL1(g),CRY1(h),CRY2(i),PER1(j),PER2(k) andSIRT1(l) gene expression. The data represent mean±s.d. of triplicate. Figure 2: Depletion of MTA1 disrupts the rhythmic expression of core clock genes. ( a , b ) MTA1 +/+ MEFs were grown to confluence in DMEM/F-12 medium containing 5% fetal bovine serum (FBS) for 6 days and shifted to medium containing 50% adult horse serum for 2 h. At time=0, the serum-rich medium was replaced with serum-free medium and cells were collected at the indicated time points for western blot analysis with the indicated antibodies ( a ) or qPCR analysis of MTA1 mRNA levels ( b ). ( c ) Protein extracts from MTA1 +/+ and MTA1 −/− MEFs were subjected to the western blot analyses with the indicated antibodies. ( d – l ) Serum-shocked MTA1 +/+ and MTA1 −/− MEFs as described above were collected at the indicated time points for qPCR analysis of MTA2 ( d ), MTA3 ( e ), CLOCK ( f ), BMAL1 ( g ), CRY1 ( h ), CRY2 ( i ), PER1 ( j ), PER2 ( k ) and SIRT1 ( l ) gene expression. The data represent mean±s.d. of triplicate. Full size image CLOCK–BMAL1 heterodimer stimulates MTA1 transcription As the MTA1 promoter contains a canonical E-box motif ( Supplementary Tables S1 and S2 ), we next examined whether the CLOCK–BMAL1 heterodimer could interact with the E-box motif at the MTA1 promoter using chromatin immunoprecipitation (ChIP)-based promoter assays. To this aim, the MTA1 promoter was subdivided into approximately four 400-bp segments according to the E-box motif position ( Fig. 3a , upper panel). Results showed that CLOCK ( Fig. 3b ) or BMAL1 ( Fig. 3c ) alone or CLOCK–BMAL1 heterodimer ( Fig. 3d ) were specifically recruited to the R3 region (from −3,096 to −2,789), but not the R1 (from −5,147 to −4,993), R2 (from −4,594 to −4,220) and R4 regions (from −1,836 to −1,442) of the MTA1 promoter ( Fig. 3a , lower panel). As the R3 region of the MTA1 promoter contains a canonical E-box motif ( Fig. 3a and Supplementary Table S1 ), we next examined whether CLOCK and BMAL1 associate with the E-box of the MTA1 promoter by electrophoretic mobility shift assay (EMSA) using wild-type or mutant E-box oligonucleotide. As shown in Fig. 3e , we found that the basal protein–MTA1 DNA complex was supershifted by the incubation of the nuclear extracts with a specific antibody against BMAL1 (lane 4) or CLOCK (lane 5) in the presence of wild-type (lanes 1–9) but not mutant E-box oligonucleotide (lanes 10–16). These results suggest that both CLOCK and BMAL1 proteins may interact with the E-box element in the MTA1 promoter. In support of this notion, co-incubation of anti-CLOCK and anti-BMAL1 antibodies resulted in the formation of further higher molecular weight protein–DNA complexes ( Fig. 3e , lane 8). In contrast, we did not observe any supershift following addition of antibodies and probes in the absence of nuclear extracts ( Supplementary Fig. 1a , lanes 6–10) as compared with the positive controls in the presence of nuclear extracts (lanes 1–5), thus underscoring the specificity of the antibodies used in the EMSA assays ( Figs. 3e and 5h ). 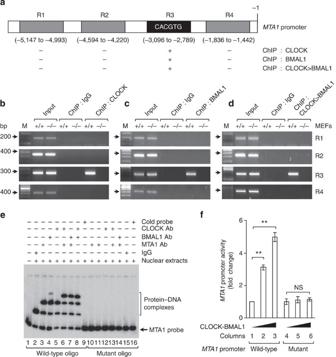Figure 3: CLOCK–BMAL1 heterodimer activates theMTA1transcription. (a) Line diagram shows the recruitment of CLOCK, BMAL1 or CLOCK–BMAL1 onto different regions onto theMTA1promoter. (b–d) ChIP analysis of recruitment of CLOCK (b), BMAL1 (c) or CLOCK–BMAL1 (d) onto theMTA1promoter. (e) EMSA analysis of the binding of CLOCK, BMAL1 or MTA1 to theMTA1promoter using nuclear extracts from MTA1+/+cells. Ab, antibody. (f) NIH3T3 cells were transfected with 100 ng of pGL3-MTA1 expression vector in the absence or presence of increasing doses of Flag-CLOCK/BMAL1 (100 and 200 ng). After 48 h of transfection, theMTA1luciferase activity was determined as described in Methods. Each column shows mean±s.d. of triplicate (Student’st-test). **P<0.01; NS, no significance. Figure 3: CLOCK–BMAL1 heterodimer activates the MTA1 transcription. ( a ) Line diagram shows the recruitment of CLOCK, BMAL1 or CLOCK–BMAL1 onto different regions onto the MTA1 promoter. ( b – d ) ChIP analysis of recruitment of CLOCK ( b ), BMAL1 ( c ) or CLOCK–BMAL1 ( d ) onto the MTA1 promoter. ( e ) EMSA analysis of the binding of CLOCK, BMAL1 or MTA1 to the MTA1 promoter using nuclear extracts from MTA1 +/+ cells. Ab, antibody. ( f ) NIH3T3 cells were transfected with 100 ng of pGL3-MTA1 expression vector in the absence or presence of increasing doses of Flag-CLOCK/BMAL1 (100 and 200 ng). After 48 h of transfection, the MTA1 luciferase activity was determined as described in Methods. Each column shows mean±s.d. of triplicate (Student’s t -test). ** P <0.01; NS, no significance. 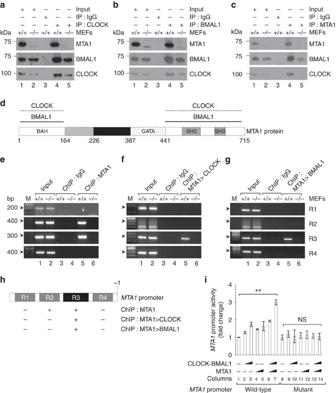Figure 4: MTA1 forms a complex with CLOCK–BMAL1 and activates its own transcription. (a–c) Nuclear extracts from MTA1+/+and MTA1−/−MEFs were subjected to immunoprecipitation (IP) analysis with an anti-CLOCK (a), anti-BMAL1 (b), anti-MTA1 (c) antibodies or control IgG, followed by western blotting with the indicated antibodies. (d) Schematic representation of the domains of MTA1 for CLOCK and BMAL1 binding. BAH, bromo-adjacent homology; GATA, GATA-type zinc-finger domain; SH3, SRC homology 3. (e–g) ChIP analysis of recruitment of MTA1 (e), MTA1–CLOCK (f) or MTA1–BMAL1 (g) onto theMTA1promoter. (h) Line diagram shows the recruitment of MTA1, MTA1–CLOCK or MTA1–BMAL1 onto different regions at theMTA1promoter. (i) NIH3T3 cells were transfected with the pGL3-MTA1 expression vector (100 ng) in the presence or absence of increasing doses of T7-MTA1 (100, 200 ng) and Flag-CLOCK/BMAL1 (100, 200 ng) alone or in combination. After 48 h of transfection, theMTA1luciferase activity was determined as described in Methods. Each column shows mean±s.d. of triplicate (Student’st-test). **P<0.01; NS, no significance. Full size image Figure 4: MTA1 forms a complex with CLOCK–BMAL1 and activates its own transcription. ( a – c ) Nuclear extracts from MTA1 +/+ and MTA1 −/− MEFs were subjected to immunoprecipitation (IP) analysis with an anti-CLOCK ( a ), anti-BMAL1 ( b ), anti-MTA1 ( c ) antibodies or control IgG, followed by western blotting with the indicated antibodies. ( d ) Schematic representation of the domains of MTA1 for CLOCK and BMAL1 binding. BAH, bromo-adjacent homology; GATA, GATA-type zinc-finger domain; SH3, SRC homology 3. ( e – g ) ChIP analysis of recruitment of MTA1 ( e ), MTA1–CLOCK ( f ) or MTA1–BMAL1 ( g ) onto the MTA1 promoter. ( h ) Line diagram shows the recruitment of MTA1, MTA1–CLOCK or MTA1–BMAL1 onto different regions at the MTA1 promoter. ( i ) NIH3T3 cells were transfected with the pGL3-MTA1 expression vector (100 ng) in the presence or absence of increasing doses of T7-MTA1 (100, 200 ng) and Flag-CLOCK/BMAL1 (100, 200 ng) alone or in combination. After 48 h of transfection, the MTA1 luciferase activity was determined as described in Methods. Each column shows mean±s.d. of triplicate (Student’s t -test). ** P <0.01; NS, no significance. 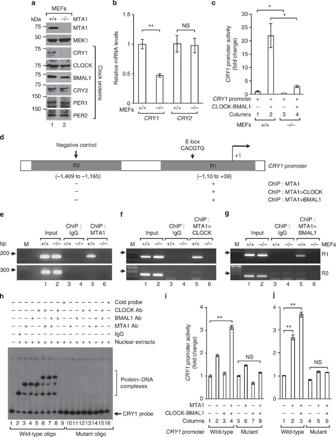Figure 5: MTA1 regulatesCRY1expression. (a) Protein extracts of MTA1+/+and MTA1−/−MEFs were subjected to western blot analysis using the indicated specific antibodies. (b) qPCR analysis ofCRY1andCRY2mRNA levels in MTA1+/+and MTA1−/−MEFs. (c) MTA1+/+and MTA1−/−cells were transfected with 200 ng of pGL3-CRY1 expression vector alone or in combination with 500 ng of Myc-CLOCK/BMAL1 plasmid DNA and theCRY1luciferase activity was determined after 48 h of transfection. (d) Line diagram shows the recruitment of MTA1, MTA1–CLOCK or MTA1–BMAL1 onto different regions at theCRY1promoter. (e–g) ChIP analysis of recruitment of MTA1 (e), MTA1–CLOCK (f) or MTA1–BMAL1 (g) onto theCRY1promoter. (h) EMSA analysis of the binding of CLOCK, BMAL1, or MTA1 to theCRY1promoter using nuclear extract from MTA1+/+cells. Ab, antibody. (i–j) NIH3T3 cells were transfected with 100 ng of pGL3-CRY1expression vector in the presence or absence 50 ng of T7-MTA1, 50 ng of Flag-CLOCK/BMAL1 alone or in combination and theCRY1luciferase activity was determined as described above. (i) Each column shows mean±s.d. of triplicate (Student’st-test). *P<0.05; **P<0.01; NS, no significance. Full size image Figure 5: MTA1 regulates CRY1 expression. ( a ) Protein extracts of MTA1 +/+ and MTA1 −/− MEFs were subjected to western blot analysis using the indicated specific antibodies. ( b ) qPCR analysis of CRY1 and CRY2 mRNA levels in MTA1 +/+ and MTA1 −/− MEFs. ( c ) MTA1 +/+ and MTA1 −/− cells were transfected with 200 ng of pGL3-CRY1 expression vector alone or in combination with 500 ng of Myc-CLOCK/BMAL1 plasmid DNA and the CRY1 luciferase activity was determined after 48 h of transfection. ( d ) Line diagram shows the recruitment of MTA1, MTA1–CLOCK or MTA1–BMAL1 onto different regions at the CRY1 promoter. ( e – g ) ChIP analysis of recruitment of MTA1 ( e ), MTA1–CLOCK ( f ) or MTA1–BMAL1 ( g ) onto the CRY1 promoter. ( h ) EMSA analysis of the binding of CLOCK, BMAL1, or MTA1 to the CRY1 promoter using nuclear extract from MTA1 +/+ cells. Ab, antibody. ( i – j ) NIH3T3 cells were transfected with 100 ng of pGL3- CRY1 expression vector in the presence or absence 50 ng of T7-MTA1, 50 ng of Flag-CLOCK/BMAL1 alone or in combination and the CRY1 luciferase activity was determined as described above. ( i ) Each column shows mean±s.d. of triplicate (Student’s t -test). * P <0.05; ** P <0.01; NS, no significance. Full size image To test whether the CLOCK–BMAL1 heterodimers could drive the transcription from the MTA1 promoter through the E-box motif, we transfected mouse NIH3T3 fibroblasts, which contain circadian oscillators and have been widely used in circadian clock studies [2] , [28] , [29] , with a minimal MTA1 promoter construct (from −3,032 to −2,427) that includes a canonical E-box motif as described previously [30] . We found that coexpression of CLOCK and BMAL1 stimulates the MTA1 promoter activity in a dose-dependent manner ( Fig. 3f , lanes 1–3). In contrast, expression of CLOCK or BMAL1 alone had limited effects on MTA1 promoter activity ( Supplementary Fig. S1b , columns 2 and 3, respectively). More interestingly, the CLOCK–BMAL1-dependent activation of the MTA1 promoter was abolished when the E-box motif was mutated ( Fig. 3f , columns 4–6). These results suggest that MTA1 is a clock-controlled gene that is transcriptionally activated by the CLOCK–BMAL1 heterodimer. MTA1 stimulates its own transcription via a positive feedback loop Given that the autoregulatory feedback loops are common features of circadian clock in animals and plants [1] , [6] , [7] , we next examined the possibility that MTA1 may influence its own transcription via interacting with the CLOCK–BMAL1 heterodimer. Indeed, immunoprecipitation (IP) of the endogenous CLOCK ( Fig. 4a ) or BMAL1 ( Fig. 4b ) protein co-precipitated the endogenous MTA1 in the nuclear extracts from the MTA1 +/+ but not from MTA1 −/− MEFs (upper panel, compare lane 4 with 5). Reciprocally, IP of the endogenous MTA1 protein also co-precipitated the endogenous CLOCK and BMAL1 proteins in the MTA1 +/+ MEFs but not in MTA1 −/− cells ( Fig. 4c , compare lane 4 with 5). These results suggest that MTA1 interacts with CLOCK and BMAL1 in vivo . To test whether MTA1 directly binds to CLOCK or BMAL1, in vitro glutathione S -transferase (GST) pull-down assays were performed using in vitro -translated, [ 35 S]-methionine-labelled BMAL1 and CLOCK and GST-tagged MTA1 deletion constructs (GST-MTA1) [31] ( Supplementary Fig. S2 ). Interestingly, we found that both BMAL1 ( Supplementary Fig. S2a ) and CLOCK ( Supplementary Fig. S2b ) proteins bound to the amino terminus (residues 1–164) and the carboxyl terminus (residues 442–715) of the MTA1 protein ( Fig. 4d ). It is interesting to note that the amino terminus of MTA1 contains a bromo-adjacent homology domain important for protein–protein interaction [32] , whereas the carboxyl terminus of MTA1 contains several Src homology domain 3-binding motifs that function as peptide- and protein-recognition modules [33] . Thus, it is conceivable that MTA1 forms a complex with the CLOCK–BMAL1 heterodimer, probably through its bromo-adjacent homology domain and Src homology domain 3-binding motifs. We next tested whether MTA1 utilizes the CLOCK–BMAL1 heterodimer to get recruited onto its own promoter using a ChIP-based promoter walk assay. Single-ChIP assay with an anti-MTA1 antibody showed that MTA1 was specifically recruited to the R2 (from −4,594 to −4,220) and R3 regions (from −3,096 to −2,789), but not the R1 (from −5,147 to −4,993) and R4 (from −1,836 to −1,441) regions, of the MTA1 promoter in the MTA1 +/+ but not in MTA1 −/− MEFs ( Fig. 4e , compare lane 5 with 6, and Fig. 4h , lower panel). Interestingly, sequential double-ChIP assay, wherein the first ChIP with an anti-MTA1 antibody was followed by a second ChIP with an anti-CLOCK ( Fig. 4f ) or anti-BMAL1 antibody ( Fig. 4g ), revealed the recruitment of the MTA1–CLOCK or MTA1–BMAL1complex onto the R3 region, but not the R1, R2 or R4 regions, of the MTA1 promoter ( Fig. 4h , lower panel). In support of these observations, a serum shock stimulated the recruitment of the MTA1–CLOCK or MTA1–BMAL1 complex onto the R3 region of the MTA1 promoter in MTA1 +/+ but not MTA1 −/− MEFs in a time-dependent manner ( Supplementary Fig. S3 , compare lanes 1–4 with 5–8). Further, EMSA assays demonstrated that the binding of the MTA1–CLOCK ( Fig. 3e , lane 6) or the MTA1–BMAL1 ( Fig. 3e , lane 7) complex to the MTA1 promoter DNA. Consistent with these results, MTA1 and CLOCK–BMAL1 synergistically stimulated the MTA1 promoter activity in a dose-dependent manner ( Fig. 4i , columns 1–7) but failed to stimulate the activity of MTA1 promoter with an E-box mutant ( Fig. 4i , columns 8–14). These results establish a positive feedback loop for MTA1 in regulating its own transcription involving the CLOCK–BMAL1 activator complex. CRY1 expression is compromised in MTA1-deficient cells We next examined whether MTA1 also regulates the expression of other components of the clock system. As shown in Fig. 5a , the levels of CRY1 protein were substantially decreased in the unsynchronized MTA1 −/− MEFs as compared with the levels in the MTA1 +/+ MEFs (compare lane 2 with 1). In contrast, no significant differences were observed in the levels of CLOCK, BMAL1, CRY2, PER1 and PER2 proteins between the unsynchronized MTA1 +/+ and MTA1 −/− cells (compare lane 2 with 1). Interestingly, the levels of mRNAs for CLOCK ( Fig. 2f ), BMAL1 ( Fig. 2g ), CRY2 ( Fig. 2i ), PER1 ( Fig. 2j ) and PER2 ( Fig. 2k ) were differentially regulated by the serum shock between the synchronized MTA1 +/+ and MTA1 −/− MEFs. The observed discordance in the expression levels of mRNAs and proteins among the synchronized versus unsynchronized MEFs is reflective of differing states of MEFs. In addition, previous studies have demonstrated that there is no linear correlation between the levels of mRNAs and proteins in biologic systems because of various biological factors such as post-translational regulatory mechanisms and the differences in mRNA and protein turnover rates [29] , [34] , [35] , [36] , [37] , [38] , [39] , [40] , [41] . In line with the changes observed for CRY1 protein levels, CRY1 mRNA levels were reduced in the unsynchronized MTA1 −/− MEFs as compared with the levels in MTA1 +/+ MEFs ( Fig. 5b ). To gain an insight into the regulation of CRY1 by MTA1, we next examined whether MTA1 affects the CRY1 promoter activity. As shown in Fig. 5c , knockout of MTA1 inhibits the basal (compare column 3 with 1) as well as the CLOCK–BMAL1-activated CRY1 promoter activity (compare column 4 with 2). We next determined the possibility of MTA1 recruitment onto the CRY1 promoter. To this end, the CRY1 promoter was subdivided into two approximate regions of 400-bp each according to the E-box motif position ( Fig. 5d , upper panel). Single ChIP with an anti-MTA1 antibody demonstrated that MTA1 was recruited to the R1 (from −110 to +39) but not the R2 region (from −1,409 to −1,165) of the CRY1 promoter in the MTA1 +/+ but not in MTA1 −/− MEFs ( Fig. 5e , compare lane 5 with 6). Sequential double-ChIP analyses demonstrated that the MTA1–CLOCK ( Fig. 5f ) or the MTA1–BMAL1 ( Fig. 5g ) complexes were also recruited to the same R1 region of the CRY1 promoter in the MTA1 +/+ but not MTA1 −/− MEFs ( Fig. 5d , lower panel). As expected, a serum shock stimulated the recruitment of the MTA1–CLOCK or MTA1–BMAL1 complexes onto the CRY1 promoter in MTA1 +/+ but not MTA1 −/− MEFs in a time-dependent manner ( Supplementary Fig. S4 , compare lanes 1–4 with 5–8). To further support these findings, we next carried out EMSA assay using the wild-type or E-box-mutant oligonucleotide probe ( Fig. 5h ). We found that the noted protein– CRY1 DNA complex was effectively retarded by the inclusion of specific antibodies against MTA1 (lane 3), BMAL1 (lane 4) or CLOCK (lane 5) only in the presence of wild-type (lanes 1–9) but not mutant E-box oligonucleotide (lanes 10–16). Further, co-incubation of antibodies against MTA1, CLOCK or BMAL1 resulted in the formation of further higher molecular weight protein–DNA complexes ( Fig. 5h , lanes 6–8). These results suggest that the MTA1–CLOCK–BMAL1 complex could bind to the CRY1 promoter through the E-box element. Consistent with these observations, MTA1 and CLOCK–BMAL1 synergistically stimulated the wild-type but not E-box-mutant CRY1 promoter activity ( Fig. 5i , compare columns 1–4 with 5–8, and Fig. 5j , compare columns 1–3 with 4–6). Collectively, these findings suggest that MTA1 protein gets recruited onto the CRY1 promoter through the CLOCK–BMAL1 activator complex and positively regulates CLOCK–BMAL1-driven CRY1 transcription. MTA1 deacetylates BMAL1 through deacetylase SIRT1 As CRY1 has an essential role in the repressive arm of the clock circuit [2] , [42] and BMAL1 acetylation facilitates repressive function of CRY1 [43] , we next examined whether MTA1 affects the acetylation status of BMAL1 protein, and thus might affect the CRY1-mediated negative feedback loop. A previous study has demonstrated that BMAL1 deacetylation is regulated by class III (SIRT1) but not classes I and II HDACs [44] . Using SIRT1-knockout MEFs as positive controls, we demonstrated that MTA1 knockout leads to an increase in the levels of acetyl BMAL1 lys538 ( Fig. 6a , compare lane 2 with 1). In contrast, there was no effect of MTA1 knockout on the levels of CLOCK, an acetyltransferase responsible for BMAL1 acetylation [43] , and BMAL1 proteins as compared with its levels in MTA1 +/+ MEFs (compare lane 2 with 1). These results suggest that MTA1 could deacetylate BMAL1 protein. 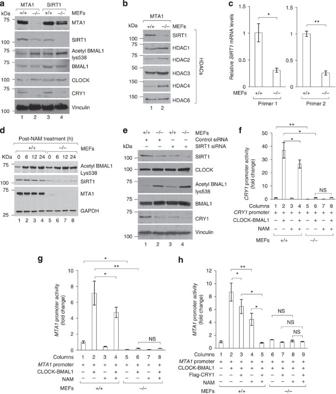Figure 6: The MTA1-SIRT1 axis is required for CLOCK–BMAL1-mediated activation of MTA1 and CRY1. (a) Protein extracts from MTA1+/+and MTA1−/−as well as SIRT1+/+and SIRT1−/−MEFs were subjected to western blot analysis with the indicated antibodies. (b) Protein extracts from MTA1+/+and MTA1−/−MEFs (the same lysates as used inFig. 2c) were subjected to western blot analysis with the indicated antibodies. (c) qPCR analysis ofSIRT1expression in MTA1+/+and MTA1−/−MEFs. (d) MTA1+/+and MTA1−/−MEFs were treated with or without 10 mM of SIRT1 inhibitor NAM for the indicated times and protein extracts were subjected to western blot analysis with the indicated antibodies. (e) MTA1+/+and MTA1−/−MEFs were transfected with control or SIRT1 siRNA. After 48 h of the second transfection, cells were subjected to western blot analysis with the indicated antibodies (the same cellular lysates were run on parallel gels). (f) MTA1+/+and MTA1−/−MEFs were transfected with 250 ng of pGL3-CRY1 expression vector in the presence or absence of 750 ng of Myc-CLOCK/BMAL1. After 24 h of transfection, cells were incubated with 10 mM nicotinamide (NAM) for another 24 h and subjected to analysis of theCRY1luciferase activities. (g) MTA1+/+and MTA1−/−MEFs were transfected with 250 ng of pGL3-MTA1 expression vector in the presence or absence of 500 ng of Myc-CLOCK/BMAL1. After 24 h of transfection, cells were incubated with 10 mM NAM for another 24 h and subjected to analysis of theMTA1luciferase activities. (h) MTA1+/+and MTA1−/−MEFs were transfected with 250 ng of pGL3-MTA1 expression vector in the presence or absence of 500 ng of Myc-CLOCK/BMAL1 or 250 ng of Flag-CRY1 alone or in combination. After 24 h of transfection, cells were incubated with 10 mM NAM for another 24 h and subjected to analysis of theMTA1luciferase activities. Each column shows mean±s.d. of triplicate (Student’st-test). *P<0.05; **P<0.01; NS, no significance. Figure 6: The MTA1-SIRT1 axis is required for CLOCK–BMAL1-mediated activation of MTA1 and CRY1. ( a ) Protein extracts from MTA1 +/+ and MTA1 −/− as well as SIRT1 +/+ and SIRT1 −/− MEFs were subjected to western blot analysis with the indicated antibodies. ( b ) Protein extracts from MTA1 +/+ and MTA1 −/− MEFs (the same lysates as used in Fig. 2c ) were subjected to western blot analysis with the indicated antibodies. ( c ) qPCR analysis of SIRT1 expression in MTA1 +/+ and MTA1 −/− MEFs. ( d ) MTA1 +/+ and MTA1 −/− MEFs were treated with or without 10 mM of SIRT1 inhibitor NAM for the indicated times and protein extracts were subjected to western blot analysis with the indicated antibodies. ( e ) MTA1 +/+ and MTA1 −/− MEFs were transfected with control or SIRT1 siRNA. After 48 h of the second transfection, cells were subjected to western blot analysis with the indicated antibodies (the same cellular lysates were run on parallel gels). ( f ) MTA1 +/+ and MTA1 −/− MEFs were transfected with 250 ng of pGL3-CRY1 expression vector in the presence or absence of 750 ng of Myc-CLOCK/BMAL1. After 24 h of transfection, cells were incubated with 10 mM nicotinamide (NAM) for another 24 h and subjected to analysis of the CRY1 luciferase activities. ( g ) MTA1 +/+ and MTA1 −/− MEFs were transfected with 250 ng of pGL3-MTA1 expression vector in the presence or absence of 500 ng of Myc-CLOCK/BMAL1. After 24 h of transfection, cells were incubated with 10 mM NAM for another 24 h and subjected to analysis of the MTA1 luciferase activities. ( h ) MTA1 +/+ and MTA1 −/− MEFs were transfected with 250 ng of pGL3-MTA1 expression vector in the presence or absence of 500 ng of Myc-CLOCK/BMAL1 or 250 ng of Flag-CRY1 alone or in combination. After 24 h of transfection, cells were incubated with 10 mM NAM for another 24 h and subjected to analysis of the MTA1 luciferase activities. Each column shows mean±s.d. of triplicate (Student’s t -test). * P <0.05; ** P <0.01; NS, no significance. Full size image As the MTA1 protein is not a putative enzyme, we next examined whether MTA1 regulates the expression of SIRT1, thus resulting in deacetylation of BMAL1. Interestingly, we found that MTA1 knockout results in a substantial reduction in the levels of SIRT1 protein ( Fig. 6a,b , compare lane 2 with 1) and mRNA ( Fig. 6c ). In contrast, MTA1 depletion did not alter the expression levels of HDAC1, 3 and 6 proteins but resulted in an easily detectable upregulation of HDAC2 and 4 ( Fig. 6b , compare lane 2 with 1). These findings suggest that MTA1 deacetylates acetylated 538 in BMAL1 through, at least in part, regulating SIRT1 expression. In support of this notion, we found that, although the basal levels of acetyl BMAL1 at Lys538 were higher in the MTA1 −/− MEFs than that in MTA1 +/+ MEFs ( Fig. 6d , compare lane 5 with 1), incubation of cells with SIRT1 inhibitor nicotinamide (NAM) [44] , [45] enhances the levels of acetyl BMAL1 lysine 538 in both MTA1 +/+ and MTA1 −/− MEFs ( Fig. 6d ). These findings suggest that SIRT1 has a functional role in the MTA1-mediated deacetylation of BMAL1. To establish a mechanistic link between the SIRT1 and BMAL1 deacetylation in the MTA1 +/+ and MTA1 −/− MEFs, we next knocked down the endogenous SIRT1 using specific SIRT1 short interfering RNAs (siRNAs) in MTA1 +/+ and MTA1 −/− MEFs. As shown in Fig. 6e , we found that MTA1 knockout leads to an increase in the levels of acetyl BMAL1 lys538 (compare lane 2 with 1), and this effect was further enhanced following depletion of SIRT1 using specific SIRT1 siRNAs (compare lane 3 with 1 and lane 4 with 2). These findings implicate a role for the MTA1-SIRT1 axis in regulating deacetylation of BMAL1 by MTA1. MTA1-SIRT1 axis is required for CRY1 activation We next investigated whether there is a functional link between the MTA1-SIRT1-BMAL1 deacetylation and the circadian clock function. Interestingly, knockdown of MTA1 resulted in a downregulation of CRY1 protein levels ( Fig. 6e , compare lane 2 with 1), and this effect was further enhanced following knockdown of the endogenous SIRT1 ( Fig. 6e , compare lane 3 with 1 and lane 4 with 2). These observations suggested that the MTA1-SIRT1 axis has a role in CRY1 regulation. In line with these findings, MTA1 knockout resulted in an appreciable reduction in the basal ( Fig. 6f , compare column 5 with 1) as well as CLOCK–BMAL1-activated CRY1 promoter activity ( Fig. 6f , compare column 2 with 6), suggesting that MTA1 is required for the CLOCK–BMAL1-mediated activation of CRY1. Further, inhibition of SIRT1 activity by the SIRT1 inhibitor NAM [44] , [45] also reduced the CLOCK–BMAL1-activated CRY1 promoter activity in the MTA1 +/+ MEFs ( Fig. 6f , compare column 4 with 2) but not in MTA1 −/− cells ( Fig. 6f , compare column 8 with 6). These results collectively suggest that the MTA1-SIRT1-BMAL1 deacetylation axis is required for CRY1 activation by CLOCK–BMAL1. MTA1-SIRT1 axis depresses CRY1-mediated repression of MTA1 As MTA1 is a positive regulator of CRY1 ( Fig. 5 ), we next examined whether the MTA1-SIRT1-BMAL1 deacetylation axis could affect MTA1 transcription by CLOCK–BMAL1. As shown in Fig. 6g , MTA1 knockout also inhibited the basal (compare column 5 with 1) as well as CLOCK–BMAL1-stimulated (compare column 6 with 2) MTA1 promoter activity. Interestingly, this effect was further enhanced by the SIRT1 inhibitor NAM [44] , [45] only in MTA1 +/+ MEFs ( Fig. 6g , compare column 3 with 1 and column 4 with 2) but not in MTA1 −/− cells ( Fig. 6g , compare column 7 with 5 and column 8 with 6). These results suggest that the MTA1-SIRT1 axis is required for CLOCK–BMAL1-mediated stimulation of MTA1 transcription. Given that the MTA1-SIRT1 axis promotes BMAL1 deacetylation ( Fig. 6a,d and e ) and acetylation of BMAL1 facilitates CRY1-mediated repression [43] , it is conceivable that the MTA1-SIRT1 axis regulates the CLOCK–BMAL1-mediated activation of MTA1 transcription, probably by derepressing CRY1-mediated negative feedback loop. To test this possibility, we next examined whether CRY1 represses CLOCK–BMAL1-mediated activation of MTA1 transcription and whether the MTA1-SIRT1 axis has any role in this process. As shown in Fig. 6h , we found that CRY1 suppresses CLOCK–BMAL1-activated MTA1 promoter activity (compare column 3 with 2), and this effect was further enhanced following inhibition of SIRT1 activity by SIRT1 inhibitor NAM in MTA1 +/+ MEFs (compare column 5 with 3) but not in MTA1 −/− cells (compare column 9 with 7). These results indicate that inhibition of SIRT1 activity by the SIRT1 inhibitor NAM results in an increased level of BMAL1 acetylation by CLOCK, which in turn facilitates CRY1-mediated repression of MTA1. Here we discovered that MTA1, a well-recognized marker for tumour invasion and metastasis [13] , is an intrinsic regulator of the mammalian molecular clock ( Fig. 7 ). Genetic depletion of MTA1 in mice affects the response of the circadian system to ambient light, as revealed by a reduced rate of re-entrainment to standard LD cycles after light-phase advancement by 6 h and an enhanced period lengthening under constant light conditions ( Fig. 1 ). Moreover, like other clock genes, the mRNA and protein expression of MTA1 shows a circadian expression pattern ( Fig. 2a,b ). Interestingly, although MTA2 and MTA3 promoters do not contain a canonical E-box motif, they do have a non-canonical E-box motif (5′-CAGCTT-3′) [22] at their promoters ( Supplementary Table S1 ), significance of which remains to be determined in the future. 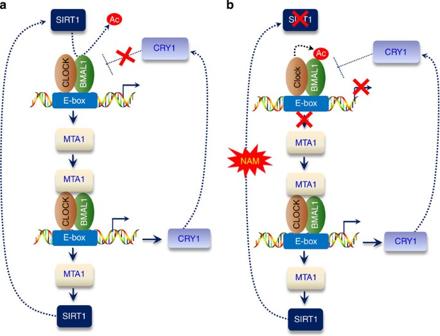Figure 7: The proposed working model. (a) The CLOCK–BMAL1 activator complex binds to the E-box element at theMTA1promoter and stimulates its transcription. MTA1, in turn, forms a complex with and recruits CLOCK–BMAL1 onto the E-box element at theMTA1andCRY1promoters, activating their expression through the E-box element at their promoters. MTA1 also regulates deacetylation of BMAL1 by regulating SIRT1 expression, resulting in derepressing CRY1-mediated transcription repression. (b) Inhibition of SIRT1 activity by the SIRT1 inhibitor NAM results in an increase in the levels of BMAL1 acetylation by CLOCK, which in turn facilitates CRY1-mediated repression of MTA1. Figure 7: The proposed working model. ( a ) The CLOCK–BMAL1 activator complex binds to the E-box element at the MTA1 promoter and stimulates its transcription. MTA1, in turn, forms a complex with and recruits CLOCK–BMAL1 onto the E-box element at the MTA1 and CRY1 promoters, activating their expression through the E-box element at their promoters. MTA1 also regulates deacetylation of BMAL1 by regulating SIRT1 expression, resulting in derepressing CRY1-mediated transcription repression. ( b ) Inhibition of SIRT1 activity by the SIRT1 inhibitor NAM results in an increase in the levels of BMAL1 acetylation by CLOCK, which in turn facilitates CRY1-mediated repression of MTA1. Full size image The emerging physiological role for MTA1 in the molecular clock is supported by several lines of evidence. First, the CLOCK–BMAL1 heterodimer activates MTA1 transcription through the conserved E-box element at its promoter ( Fig. 3f ). Second, MTA1 is a bona fide binding partner of the CLOCK–BMAL1 complex ( Fig. 4a–d and Supplementary Fig. S2 ) and recruits CLOCK–BMAL1 onto its own promoter and simulates its transcription ( Fig. 3 ), thus establishing a positive feedback loop between MTA1 and CLOCK–BMAL1. Third, MTA1 is required for transcriptional stimulation of CRY1 by CLOCK–BMAL1 ( Fig. 5 ), and CRY1, in turn, inhibits the CLOCK–BMAL1-mediated stimulation of MTA1 transcription ( Fig. 6h ), thus establishing another feedback loop between MTA1 and CRY1. Finally, MTA1 deacetylates BMAL1 at lysine 538 by regulating SIRT1 expression ( Fig. 6a–e ), and the MTA1-SIRT1-BMAL1 deacetylaiton axis is involved in the CLOCK–BMAL1-mediated activation of MTA1 and CRY1, probably by depressing CRY1-mediated negative feedback loop ( Figs 6f–h and 7a ). Together, these findings establish that MTA1 functions in the positive limb of the clock machinery at multiple levels and is an important component of an additional autoregulatory feedback loop with interlocks with the core feedback loop of circadian oscillation. As expected, this study also raises several interesting questions to be answered in future research. Given that clock disruption by environmental or genetic factors has been implicated in human cancer [46] , [47] and that many of clock genes are related to regulatory mechanisms that are important in cancer [48] , understanding whether and how perturbation of the physiological function of MTA1 in circadian clock are connected to its oncogenic activity in tumour progression will be the central topic of future studies. In addition, the transcriptional activator CLOCK could acetylate histones and non-histone substrates that are crucial for the circadian machinery [43] , [49] , [50] . It would be of interest to examine whether CLOCK could target its binding partner MTA1 for acetylation, which in turn controls its function in circadian clock in the near future. In conclusion, we demonstrated that MTA1 is a component of the circadian clock that regulates the CLOCK–BMAL1-mediated positive limbs. These findings broaden our understanding of the physiological functions and underlying mechanisms of MTA1 in mammalian physiology and behaviour and would be a starting point for investigating the missing molecular link between deregulation of the circadian clock and tumour progression. Animals and cell culture MTA1-knockout (MTA1 −/− ) mice were generated in our laboratory by deleting exon 2 of MTA1 gene and maintained at C57/BL6 and 129sv mixed genetic background [51] , [52] . Wild-type and MTA1 −/− male and female mice were housed under a 12/12 LD cycle unless otherwise noted with food and water ad libitum . All animal studies were conducted in accordance with the regulations of the committees on Animal Care and Use at the University of Texas M.D. Anderson Cancer Center and the University of Houston (Houston, TX). MEFs derived from either MTA1 +/+ or MTA1 −/− mice were generated by collecting embryos at embryonic day 9 [51] and maintained thereafter. SIRT1 +/+ and SIRT1 −/− MEFs [53] were kindly provided by Dr Chu-Xia Deng (National Institutes of Health, Bethesda, MD). Cells were grown in DMEM/Ham’s F-12 supplemented with 10% fetal bovine serum and 1 × antibiotic-antimycotic solution (Invitrogen, Carlsbad, CA). To perform the serum-shock studies [27] , MTA1 +/+ and MTA1 −/− MEFs were cultured in medium containing 5% fetal bovine serum for 4 days to reach confluence. After 2 days of confluences, the cells were treated with 50% horse serum (Invitrogen) for 2 h. At time=0, the medium was replaced by serum-free medium. At the indicated time points, cells were washed once with ice-cold PBS and collected for further analysis. Circadian activity rhythms Circadian wheel-running experiments ( Fig. 1 ) were conducted in the Animal Facility at the University of Houston as described previously [25] , [54] . Briefly, MTA1 +/+ and MTA1 −/− male and female mice (the numbers of males and females used for each experiments are described in the figure legend of Fig. 1 ) at the age of 6–10 weeks were quarantined in group cages for 10 days under 12/12 LD cycles (lights on at 0700 hours). After release from quarantine, mice were individually housed in cages equipped with running wheels in ventilated, light-tight chambers with controlled lighting, entrained to a 12/12 LD cycle (lights on at 0700 hours in central standard time; 100–150 lux) for at least 3 weeks. After stable entrainment was apparent, groups of MTA1 +/+ and MTA1 −/− mice were exposed to either constant darkness or constant light (150 lux) for at least 4 weeks. Activity was recorded using the ClockLab data collection system (Actimetrics, Wilmette, IL) and free-running period ( τ ) was determined by Periodogram analysis of 400 continuous hours of wheel-running data collected from animals maintained under DD or LL. To determine the rates of re-entrainment to a 12/12 LD cycle, groups of MTA1 +/+ and MTA1 −/− maintained on 12/12 LD dark cycles for at least 3 weeks were subjected to a 6-h phase advance of the LD cycle. This was achieved by truncating the dark phase on a single cycle by 6 h. Activity rhythms were followed for an additional 20 days after the phase shift. The number of days required for stable re-entrainment to the 6-h phase advance was determined by fitting a straight line through activity onsets on days 10–20 after the phase shift and counting the number of activity onsets that occurred between the day of the phase shift and the first two consecutive onsets that fell on this line. Expression vectors and transfection Flag-tagged mCLOCK and mBMAL1 pcDNA3.1 expression constructs (Flag-mClock and Flag-mBmal1, respectively) were provided by Kazuhiro Yagita (Nagoya University Graduate School of Science, Nagoya, Japan) [55] . Myc-CLOCK and Myc-BMAL1 were kindly provided by Paolo Sassone-Corsi [43] (University of California, Irvine, CA). The pGL3-mCry1-luciferase expression vector was kindly provided by Roman V. Kondratov (Lerner Research Institute, Cleveland Clinic, Cleveland, OH) [56] . Cloning and characterization of the pGL3-mMTA1-luciferase expression vectors [30] , GST-MTA1 deletion constructs [31] and pcDNA3.1-MTA1 expression vector [20] have been described previously. Mutagenesis of E-box element (mutate 5′-CACGTG-3′ to 5′-GCGCGC-3′) in pGL3-mCry1 and pGL3-mMTA1 expression vectors were carried out using a Stratagene QuikChange site-directed mutagenesis kit (Stratagene, La Jolla, CA) using the designed primers ( Supplementary Table S3 ) and confirmed by DNA sequencing. ON-TARGETplus SMARTpool specific siRNAs targeting mouse SIRT1 were purchased from Dharmacon (Lafayette, CO). Plasmid DNA was purified using QIAGEN Plasmid Midi Kit (QIAGEN, Valencia, CA) and transfections were carried out using FuGENE HD Transfection Reagent (Roche Applied Science, Indianapolis, IN) according to the manufacturer’s instructions. Cells were co-transfected with the indicated vectors, and the total amount of DNA was maintained equal with corresponding empty vectors [57] . The transfection of siRNA was performed twice at 24-h intervals with Oligofectamine reagent (Invitrogen) following the manufacturer’s protocol. Cells were subjected to further analyses after 48 h of the second transfection [57] . Western blot and IP Sources of antibodies were as following: rabbit polyclonal anti-MTA1, anti-MTA2, anti-MTA3 and anti-BMAL1 (Bethyl Laboratories, Montgomery, TX), rabbit polyclonal anti-PER1 and anti- acetyl BMAL1 (Lys538; Millipore, Billerica, MA), mouse monoclonal anti-vinculin (hVIN-1), anti-actin (AC-40), rabbit polyclonal anti-HDAC4 (DM-15; Sigma-Aldrich, St. Louis, MO), rabbit monoclonal anti-CLOCK (D45B10), anti-SIRT1(D60E1), anti-HDAC6(D21B10), mouse monoclonal anti-MEK1 (61B12; Cell Signaling Technology, Danvers, MA), rabbit polyclonal anti-PER2 (H-90), anti-HDAC2 (H-54), anti-HDAC3 (H-99), mouse monoclonal anti-CRY1 (W-L5), goat polyclonal anti-HDAC1 (C-19) and anti-BMAL1 (N-20; Santa Cruz Biotechnology, Santa Cruz, CA), rabbit polyclonal anti-CRY1, anti-CRY2 and mouse monoclonal anti-histone H3 (acetyl K9; Abcam, Cambridge, MA). Mouse monoclonal anti-GAPDH antibody was kindly provided by Dr Ferid Murad laboratory (George Washington University, Washington, DC). All primary antibodies for western blot and IP analyses were used according to the recommended dilution by manufacturers’ instructions. Horseradish peroxidase-conjugated secondary antibodies and enhanced chemiluminescence reagents were purchased from Amersham Biosciences (Piscataway, NJ). The Trueblot IP beads and secondary antibodies were obtained from Rockland Immunochemicals Inc (Gilbertsville, PA). Protein extracts, western blot and IP analysis were carried out as described previously [57] . Briefly, total cellular lysates were prepared by lysing the cells with radioimmunoprecipitation assay buffer containing 1 × protease inhibitor cocktail (Roche Applied Science) and 1 × phosphatase inhibitor cocktail I and II (Sigma-Aldrich), and were then resolved by SDS–PAGE, transferred to nitrocellulose membranes and incubated with the indicated antibodies. Signal detections were performed using enhanced chemiluminescence reagents [57] . Nuclear extracts were prepared using high salt extraction method [58] . For IP analysis, the nuclear lysates were incubated with 1 μg of primary antibody and corresponding control IgG overnight at 4 °C on a rocker platform, followed by incubation with total 30 μl of Trueblot IP beads (Rockland Immunochemicals Inc) for 2 h at 4 °C. Bead-bound immunocomplexes were washed with washing buffer for three to five times to eliminate non-specific binding, and then dissolved in a sample buffer for SDS–PAGE. To reduce interference by the ~55 kDa heavy and ~23 kDa light chains of the immunoprecipitating antibody, horseradish peroxidase-conjugated TrueBlot secondary antibodies (Rockland Immunochemicals Inc) were used in the IP/immunoblotting applications [57] . Full gel scans can be found in Supplementary Fig. S5 . Promoter analysis Cells were seeded on a six-well plate and transfected the following day with the indicated expression vectors using FuGENE HD Transfection Reagent (Roche Applied Science) [18] . Empty vector was used to equalize the amount of plasmid DNA for each transfection. After 48 h of transfection, cells were assayed for β-gal activity (Tropix Galacton-Star system, Applied Biosystem) and luciferase activity (Luciferase Assay System, Promega, Madison, WI) using a luminometer (Berthold Technologies) according to the manufacturer’s protocol [18] . For each sample, luciferase activity was normalized by determining luciferase/β-gal activity ratios and averaging the values from triplicate wells. Statistical analysis was performed by a Student’s t -test for unpaired samples. Quantitative real-time PCR For quantitative real-time PCR (qPCR) analysis, total RNA was isolated by using Trizol reagent (Invitrogen), and first-strand cDNA synthesis was carried out with SuperScript II reverse transcriptase (Invitrogen) using 2 μg of total RNA and oligo (dT) primer [18] . The resultant cDNA was subjected to qPCR by using the iQTM SYBR Green Supermix (Bio-Rad Laboratories, Hercules, CA) on a CFX96 Real-Time PCR Detection System (Bio-Rad Laboratories) [18] . The values for specific genes were normalized to housekeeping controls. All of qPCR primers were synthesized by Sigma-Aldrich and the sequences of the primers are available in Supplementary Table S4 . ChIP assay The ChIP assays were performed using the ChIP Assay Kit (Millipore, Billerica, MA) according to the manufacturer’s instructions [18] . Briefly, cells were crosslinked with 1% formaldehyde for 10 min at 37 °C. The sonicated chromatin materials were immunoprecipiated with the indicated antibodies (1–3 μg of antibody in 1 ml of chromatin solution) at 4 °C overnight. The resulting DNA fragments were purified and subjected to PCR analysis using primers listed in Supplementary Tables S5 and S6 . Full gel scans can be found in Supplementary Fig. S5 . Electrophoretic mobility shift assay Nuclear extracts were prepared using a Nonidet P-40 lysis method [58] and 2 μg of nuclear extracts was used for each reaction [18] . EMSA for MTA1 or CRY1 promoter binding was performed using the annealed [γ- 32 P] ATP end-labelled oligonucleotides in a 20-μl reaction mixture for 15 min at 20 °C. Samples were run on a non-denaturing 5% polyacrylamide gel and imaged by autoradiography. Specific competitions were performed by adding a 100-fold excess of cold probe to the incubation mixture, and supershift EMSAs were performed by adding about 1 μg of the indicated antibodies. GST pull-down assay GST-fused recombinant proteins were expressed in Escherichia coli BL21 and purified using glutathione sepharose 4B (GE Healthcare, Piscataway, NJ) [18] . In vitro -translated proteins were produced using the TNT T7 Quick Coupled Transcription/Translation System (Promega) in the presence of L -[ 35 S]-methionine (PerkinElmer, Waltham, MA) according to the manufacturer’s protocol [18] , and then incubated with GST-MTA1 or GST protein on glutathione sepharose in a 1-ml binding buffer (20 mM Tris–HCl, pH 8.0, 50 mM NaCl, 10% glycerol and 0.1% NP-40) at 4 °C overnight. After washing sepharose with binding buffer three times, proteins were analysed on SDS–PAGE. How to cite this article: Li, D.-Q. et al. Metastasis-associated protein 1 is an integral component of the circadian molecular machinery. Nat. Commun. 4:2545 doi: 10.1038/ncomms3545 (2013).